Redefining the concept of protease-activated receptors: cathepsin S evokes itch via activation of Mrgprs Sensory neurons expressing Mas-related G-protein-coupled receptors (Mrgprs) mediate histamine-independent itch. We show that the cysteine protease cathepsin S activates MrgprC11 and evokes receptor-dependent scratching in mice. In contrast to its activation of conventional protease-activated receptors, cathepsin S-mediated activation of MrgprC11 did not involve the generation of a tethered ligand. We demonstrate further that different cysteine proteases selectively activate specific mouse and human Mrgpr family members. This expansion of our understanding by which proteases interact with G-protein-coupled receptors (GPCRs) redefines the concept of what constitutes a protease-activated receptor. The findings also implicate proteases as ligands to members of this orphan receptor family while providing new insights into how cysteine proteases contribute to itch. The sensation of itch is relayed from the skin to the brain via a complex but orchestrated series of signals. Itch is initiated when exogenous or endogenous pruritogens activate receptors or channels on the peripheral projections of primary sensory neurons, the cell bodies of which reside in the dorsal root or trigeminal ganglia. Specific members of the family of Mas-related G-protein-coupled receptors (Mrgprs) are expressed by a subset of nociceptive fibres [1] . These receptors have been shown to bind select pruritogens in the periphery and mediate non-histaminergic itch [2] , [3] . For example, mouse MrgprA3 and human MRGPRX1 respond to chloroquine, an anti-malarial drug, and are responsible for relaying chloroquine-induced scratching in mice [2] , [4] . Mouse MrgprC11 and human MRGPRX1 respond to a different subset of pruritogens including bovine adrenal medulla peptide (BAM8–22). MrgprC11 is activated by SLIGRL and SLIGKV, the tethered ligand peptides of respective mouse and human protease-activated receptor-2 (PAR2), while MRGPRX2 is activated by SLIGKV [2] , [3] , [5] , [6] . Trypsin, a serine protease and conventional activator of PARs, does not activate Mrgprs [3] , [7] . In addition, β-alanine, a body-building supplement known to cause itch upon ingestion, activates the MrgprD receptor expressed by nociceptive fibres [8] . In transgenic mice in which a cluster of Mrgprs has been ablated, cutaneous exposure to these pruritogens evokes significantly less scratching compared with wild-type (WT) controls. These findings underscore the importance of this family of receptors to peripheral detection of non-histaminergic itch stimuli and the subsequent activation of itch-specific neural pathways. While several exogenous compounds trigger Mrgpr activation, endogenous ligands or modulators of MrgprA3 and MrgprC11 receptors have yet to be identified. Both serine and cysteine proteases have been implicated in triggering itch and inflammation in the skin. The plant cysteine protease mucunain, derived from the tropical bean plant commonly known as cowhage, and the human cysteine protease, cathepsin S (cat S), elicit itch in human volunteers [9] , [10] . We demonstrated previously that cat S, mucunain and other plant cysteine proteases including papain, bromelain and ficin are capable of activating PAR2 and PAR4 (refs 10 , 11 ). It has been presumed that cysteine protease-evoked itch was induced via PAR2 activation. The possibility that activation of receptors other than PARs could be responsible for this sensation has not been investigated. MrgprC11 is activated by SLIGRL, a synthetic peptide generated based on the tethered sequence of the PAR2 N terminus following cleavage by serine proteases [3] . This observation is surprising because Mrgprs are not members of the PAR family. MrgprC11 does not have either arginine or lysine residues in its N-terminal extracellular domain. This receptor would neither be cleaved nor in theory activated, by serine proteases including trypsins and kallikreins. In contrast, the MrgprC11 receptor N terminus contains glycine and leucine residues, both cleavage targets for aspartyl and cysteine proteases [12] . Here, we formally investigated whether select cysteine proteases are capable of cleaving and activating MrgprC11 receptors in vitro , and determined the significance of MrgprC11 signalling in mediating cat S-induced scratching in vivo . The results demonstrate that cathepsin S provokes itching by cleavage of MrgprC11 at a specific site, resulting in activation of this receptor without generating either a tethered or diffusible ligand. Although cathepsin S can activate PAR2 receptors, such an activation is not necessary for itching provoked by this protease. Hybrid receptors in which the N terminus of MrgprC11 was replaced with the N terminus from either the β2AR or MC1R were also activated by cathepsin S. These findings highlight the possibility that cysteine proteases may exert effects on other ‘non-PAR’ GPCRs and further suggest that proteases are capable of modulating GPCRs by multiple mechanisms. Cysteine proteases cleave the N terminus of MrgprC11 MrgprC11 plays a critical role in mediating pruriception from the periphery. These receptors are known to bind several well-recognized pruritogens, including peptides resulting from the cleavage of PARs. Whether or not proteases have any direct effect on Mrgpr receptors was not known. To address this possibility, we asked whether cysteine proteases could cleave the extracellular N-terminal portion of MrgprC11. HeLa cells were transfected with a construct encoding MrgprC11 tagged with Gaussia luciferase at its N terminus and then treated with cat S or papain. Receptor cleavage was assessed by measuring levels of luminescence in the supernatants ( Fig. 1 ). Both papain and cat S induced cleavage of the MrgprC11 N terminus as determined by luminescence ( Fig. 1a ). Incubation with E-64, an irreversible cysteine protease inhibitor, blocked protease-mediated cleavage of the N termini. In separate studies, tagged MrgprC11-tranfected cells were treated with cysteine proteases. Western blots of supernatants probed with an anti- G. luciferase antibody revealed a dense band at ∼ 20 kDa in cells treated with cat S or papain, consistent with the mass expected of an N-terminal peptide tagged with G. luciferase ( Fig. 1b ). As expected, no bands were identified in controls in which transfected cells were not treated with protease. These results reveal that cysteine proteases cleave the N-terminal portion of MrgprC11. 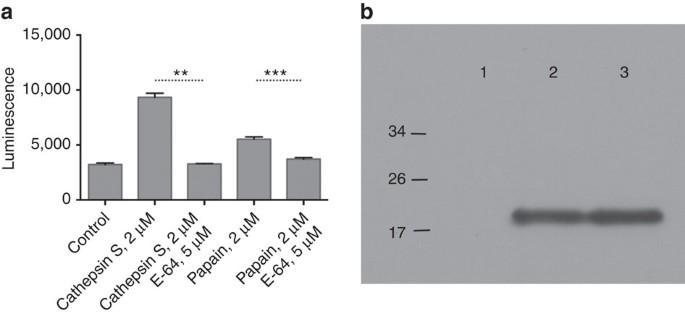Figure 1: Cysteine proteases cleave near the N terminus of MrgprC11. (a) Luminescence was measured after treating LucMrgprC11-transfected HeLa cells with cat S (2 μM) and papain (2 μM) in the presence or absence of E-64 (5 μM). Baseline luminescence has been subtracted. The data are presented as mean±s.e.m. **P<0.001, ***P<0.0005; two-tailed unpairedt-test from a representative experiment that was performed three times. (b) Western blot of LucMrgprC11 N-terminal cleavage products following treatment of transfected HeLa cells with control buffer without proteases (lane 1), papain, 0.02 μM (lane 2) and cat S, 2 μM (lane 3). The lesser amount of luminescence from papain as compared with cat S inais likely a result of higher enzyme activity and a broader range of cleavage sites for papain. Similarly, forb, a lesser concentration of papain as compared with cat S was used for incubation times to be the same for detection of luciferase. See the Methods and Discussion sections for additional comments. The LucMrgprC11 construct was functionally active (Supplementary Fig. 1). Figure 1: Cysteine proteases cleave near the N terminus of MrgprC11. ( a ) Luminescence was measured after treating LucMrgprC11-transfected HeLa cells with cat S (2 μM) and papain (2 μM) in the presence or absence of E-64 (5 μM). Baseline luminescence has been subtracted. The data are presented as mean±s.e.m. ** P <0.001, *** P <0.0005; two-tailed unpaired t -test from a representative experiment that was performed three times. ( b ) Western blot of LucMrgprC11 N-terminal cleavage products following treatment of transfected HeLa cells with control buffer without proteases (lane 1), papain, 0.02 μM (lane 2) and cat S, 2 μM (lane 3). The lesser amount of luminescence from papain as compared with cat S in a is likely a result of higher enzyme activity and a broader range of cleavage sites for papain. Similarly, for b , a lesser concentration of papain as compared with cat S was used for incubation times to be the same for detection of luciferase. See the Methods and Discussion sections for additional comments. The LucMrgprC11 construct was functionally active ( Supplementary Fig. 1 ). Full size image Cysteine proteases activate MrgprC11 in vitro We next asked whether cysteine proteases were capable of activating MrgprC11. This receptor signals via Gq, resulting in phospholipase C activation and, via second messenger recruitment, increased intracellular free Ca2+ and protein kinase C activation [4] . To assess receptor activation, we performed calcium imaging using the ratiometric calcium indicator Fura-2 in HeLa cells transfected with MrgprC11 following treatment with cat S or papain. Each protease elicited calcium responses ( Fig. 2a ), activating MrgprC11 in a concentration-dependent manner with an effector concentration for half-maximum response of ∼ 140 nM ( Fig. 2b ). Calcium responses were ablated when cells were treated with the protease inhibitor E-64 ( Fig. 2a ). In contrast to the robust responses induced by cysteine proteases, we confirmed that trypsin, a serine protease, does not activate MrgprC11 (ref. 3 ). Western blotting revealed PKC phosphorylation at serine 660 (Ser660) following treatment with cat S and papain ( Fig. 2c ). Quantification of the bands revealed an approximate 4.6-fold increase in p-PKC associated with protease activation relative to controls ( Supplementary Fig. 3 ). 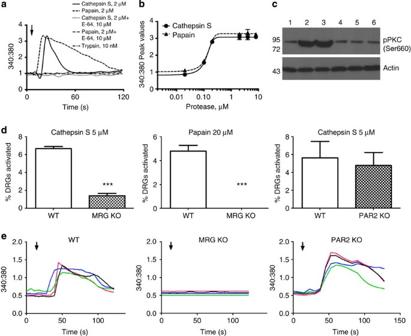Figure 2: Cysteine proteases activate MrgprC11 in heterologous cells and DRG neurons and induce PKC phosphorylation. (a) Single-cell calcium imaging in HeLa cells transfected with MrgprC11 cDNA following treatment with cat S (2 μM, solid line), papain (2 μM, dashed line), cat S+E-64 (10 μM; dotted line), papain+E-64 (10 μM; dash-dotted line) and trypsin (10 nM) dash-double-dotted line. The concentration of trypsin is typical of that used in studies of PARs. Higher concentrations of trypsin, including those in the micromolar range, did not activate MrgprC11. Additional calcium responses are detailed inSupplementary Fig. 2. (b) Concentration–effect curves for protease agonists cat S (squares) and papain (circles) on MrgprC11. Error bars represent ± s.e.m. from three sets of experiments. (c) Phosphorylation of serine 660 as a measure of second messenger is revealed by western blot. HeLa cells were transfected with MrgprC11 (lanes 1–3), or non-transfected HeLa cells (lanes 4–6) were treated with buffer alone (lanes 1 and 4), cat S (lanes 2 and 5) or papain (lanes 3 and 6). Band quantification and full scans of the blots are provided inSupplementary Fig. 3. (d) The percentage of DRG neurons activated by cat S (5 μM) was significantly reduced inMrgpr cluster knockoutmice as compared with WT DRG neurons (n=3,P<0.001). The percentage of DRG neurons activated by papain (20 μM) was reduced to zero inMrgpr cluster knockoutmice as compared with WT mice (n=3, ***P<0.001; two-tailed unpairedt-test). The percentage of DRG neurons activated by cat S (5 μM) is not significantly different between WT andPAR2−/−mice (n=3,P=0.74). (e) Representative calcium traces of cat S (5 μM) in DRG neurons from WT,Mrgpr cluster Δ−/−andPAR2−/−mice. Each trace represents responses from a single neuron. Arrows indicate application of cat S. Figure 2: Cysteine proteases activate MrgprC11 in heterologous cells and DRG neurons and induce PKC phosphorylation. ( a ) Single-cell calcium imaging in HeLa cells transfected with MrgprC11 cDNA following treatment with cat S (2 μM, solid line), papain (2 μM, dashed line), cat S+E-64 (10 μM; dotted line), papain+E-64 (10 μM; dash-dotted line) and trypsin (10 nM) dash-double-dotted line. The concentration of trypsin is typical of that used in studies of PARs. Higher concentrations of trypsin, including those in the micromolar range, did not activate MrgprC11. Additional calcium responses are detailed in Supplementary Fig. 2 . ( b ) Concentration–effect curves for protease agonists cat S (squares) and papain (circles) on MrgprC11. Error bars represent ± s.e.m. from three sets of experiments. ( c ) Phosphorylation of serine 660 as a measure of second messenger is revealed by western blot. HeLa cells were transfected with MrgprC11 (lanes 1–3), or non-transfected HeLa cells (lanes 4–6) were treated with buffer alone (lanes 1 and 4), cat S (lanes 2 and 5) or papain (lanes 3 and 6). Band quantification and full scans of the blots are provided in Supplementary Fig. 3 . ( d ) The percentage of DRG neurons activated by cat S (5 μM) was significantly reduced in Mrgpr cluster knockout mice as compared with WT DRG neurons ( n =3, P <0.001). The percentage of DRG neurons activated by papain (20 μM) was reduced to zero in Mrgpr cluster knockout mice as compared with WT mice ( n =3, *** P <0.001; two-tailed unpaired t -test). The percentage of DRG neurons activated by cat S (5 μM) is not significantly different between WT and PAR2 −/− mice ( n =3, P =0.74). ( e ) Representative calcium traces of cat S (5 μM) in DRG neurons from WT, Mrgpr cluster Δ −/− and PAR2 −/− mice. Each trace represents responses from a single neuron. Arrows indicate application of cat S. Full size image We next assessed whether cysteine proteases activate endogenously expressed Mrgpr receptors on dorsal route ganglion (DRG) neurons. Both cat S and papain treatment evoked calcium signals in DRGs from WT mice ( Fig. 2d ). Fewer DRG neurons harvested from mice in which a cluster of Mrgpr genes, including MrgprC11 , have been deleted ( Mrgpr cluster Δ −/− mice ), responded to cat S ( Fig. 2d ). The lack of response of these neurons to papain is likely due to receptor inactivation by papain under the conditions used. Because cat S is known to activate PAR2 when it is expressed in heterologous cell lines [11] , we evaluated the effect of cat S on DRGs harvested from PAR2 −/− mice. Of note, calcium responses to cat S remained intact in the absence of PAR2 receptors ( Fig. 2d ) These data support a role for protease-induced MrgprC11 activation in DRGs and, importantly, identify cat S as a potential endogenous and relevant ‘ligand’ for this receptor. The average diameter of responsive neurons was 19.3 μm, comparable to that reported previously for Mrgpr-expressing itch neurons. RNA interference (RNAi) knockdown of MrgC11 and closely related MrgprA3 was performed in DRG neurons ( Fig. 3 ). Messenger RNA levels of both genes were significantly lower as confirmed by real-time PCR ( Fig. 3d ). Knockdown of MrgprC11 only abolished the calcium response to the MrgprC11 ligand cat S but not the MrgprA3 ligand chloroquine. In contrast, knockdown of MrgprA3 only affected the response to chloroquine but not the response to cat S, showing effectiveness and specificity of RNAi. Note that transient knockdown of MrgprC11 totally abolished the cat S-induced response, while knockdown of MrgprA3 only reduced the response to chloroquine. This result is consistent with the stronger knockdown effect of MrgprC11. The observation that transient knockdown eliminates the calcium response to cat S suggests that the remaining calcium response in Mrgpr cluster knockout (KO) mice may be due to an otherwise unspecified compensation mechanism in the permanent KO. In summary, these data support a role for protease-induced MrgprC11 activation in DRGs and, importantly, identify cat S as a potential endogenous and relevant ‘ligand’ for this receptor. 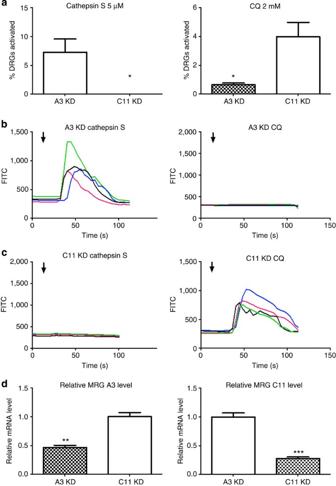Figure 3: Acute knockdown of MrgprC11 abolishes DRG response to cathepsin S. (a) MrgprA3 knockdown DRG neurons responded normally to cat S (5 μM), while MrgprC11 knockdown DRG neurons showed no response (n=4,P<0.05). In contrast, chloroquine (CQ) (2 mM) induces calcium responses in∼4% of MrgprC11 knockdown DRGs, while knockdown of MrgprA3 markedly reduced the response to CQ (n=4,P<0.05). (b) Representative calcium traces from MrgprA3 knockdown DRG neurons in response to cat S and chloroquine. (c) Representative calcium traces from MrgprC11 knockdown DRG neurons in response to cat S and chloroquine. Each trace represents responses from a single neuron. Arrows indicate application of cat S. (d) Relative messenger RNA (mRNA) level of MrgprA3 and MrgprC11 in the respective knockdown DRGs as determined by real-time PCR. The data are presented as mean±s.e.m. *P<0.05, **P<0.01; ***P<0.001; two-tailed unpairedt-test. Figure 3: Acute knockdown of MrgprC11 abolishes DRG response to cathepsin S. ( a ) MrgprA3 knockdown DRG neurons responded normally to cat S (5 μM), while MrgprC11 knockdown DRG neurons showed no response ( n =4, P <0.05). In contrast, chloroquine (CQ) (2 mM) induces calcium responses in ∼ 4% of MrgprC11 knockdown DRGs, while knockdown of MrgprA3 markedly reduced the response to CQ ( n =4, P <0.05). ( b ) Representative calcium traces from MrgprA3 knockdown DRG neurons in response to cat S and chloroquine. ( c ) Representative calcium traces from MrgprC11 knockdown DRG neurons in response to cat S and chloroquine. Each trace represents responses from a single neuron. Arrows indicate application of cat S. ( d ) Relative messenger RNA (mRNA) level of MrgprA3 and MrgprC11 in the respective knockdown DRGs as determined by real-time PCR. The data are presented as mean±s.e.m. * P <0.05, ** P <0.01; *** P <0.001; two-tailed unpaired t -test. Full size image Cathepsin S induces scratching via MrgprC11 Cat S has been shown previously to cleave and activate PAR2 in vitro [11] . It has been assumed, but never demonstrated clearly, that PAR2 activation is the mechanism by which cat S evokes scratching in mice and itch in humans [11] . However, in light of our in vitro findings that cat S-induced calcium signalling in DRGs requires MrgprC11 but not PAR2, we sought to determine the relative importance of these two receptors, if any, to cat S-induced scratching in vivo . We thus compared behavioural scratching responses with intradermal injection of cat S using the mouse cheek model in WT, Mrgpr cluster Δ −/− mice and PAR2 −/− mice. Pain and itch can be readily distinguished using the cheek injection model [13] . We only observed itch associated hind-paw scratching, but not pain-related fore-paw wiping. Injection of cat S elicited robust scratching behaviour in WT mice, but was markedly reduced in Mrgpr cluster Δ −/− mice ( Fig. 4a ). Perhaps surprisingly, scratching in PAR2 −/− mice was as robust as in WT littermates ( Fig. 4b ). These experiments underline the pivotal role of MrgprC11 in mediating cysteine protease-induced itch. 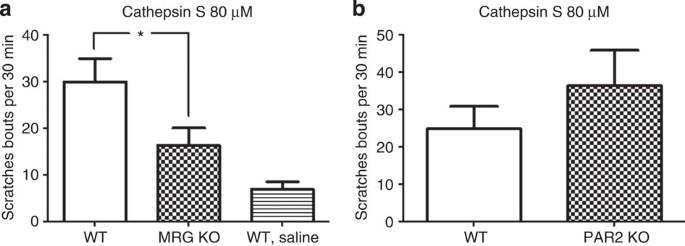Figure 4: Cathepsin S-induced scratching is reduced inMrgpr cluster Δ−/−mice. (a) Scratching behaviour of WT andMrgpr cluster Δ−/−mice in response to cat S,n=11,P=0.04, and compared with baseline saline vehicle alone (n=9). (b) Scratching behaviour of WT andPAR2−/−mice in response to cat S was not significantly different,n=7,Pvalue 0.32. The data are presented as mean±s.e.m. *P<0.05; two-tailed unpairedt-test. Figure 4: Cathepsin S-induced scratching is reduced in Mrgpr cluster Δ −/− mice. ( a ) Scratching behaviour of WT and Mrgpr cluster Δ −/− mice in response to cat S, n =11, P =0.04, and compared with baseline saline vehicle alone ( n =9). ( b ) Scratching behaviour of WT and PAR2 −/− mice in response to cat S was not significantly different, n =7, P value 0.32. The data are presented as mean±s.e.m. * P <0.05; two-tailed unpaired t -test. Full size image MrgprC11 N-terminal cleavage sites We next sought to determine whether cleavage of the extracellular N-terminal domain of MrgprC11 is necessary for protease-induced receptor activation, and if so, to identify the relevant cleavage sites. As per the MEROPS database, preferred amino acids for cleavage by cat S and papain include leucine at P2 and glycine, serine and aspartic acid at P1. Using site-specific mutagenesis, we generated a series of single-, double- and triple-substitution mutants near the MrgprC11 N terminus ( Table 1 ; Supplementary Information Note 1 ). Calcium imaging of HeLa cells transfected with these mutant receptors revealed that leucine [13] was a critical residue for cat S-mediated cleavage and activation. Papain required both aspartic acid [9] and leucine [13] for receptor cleavage and activation ( Table 1 ; Supplementary Table 1 ). None of the other candidate residues including glycine [14] , serine [6] , [7] , [15] and leucine [16] were required for receptor activation by either protease. Table 1 Responses of wild-type MrgprC11 or MrgprC11 N-terminal mutants following treatment with cat S, papain or SLIGRL as determined by calcium imaging. Full size table To determine the specific protease cleavage sites, a peptide corresponding to the 28N-terminal residues of MrgprC11 was synthesized, MDPTISSHD 9 TESTPL 13 NETGHPNCTPILT. The aspartic and leucine residues required for papain and cat S activity are indicated. This peptide was incubated with cat S or papain and then subjected to mass spectrometry (MS)/MS peptide sequence analysis, as described in Supplementary Table 1 and Note 1 , as we have done previously with cat S and PAR2 (ref. 17 ). Cat S cleavage occurred between N 16 and E 17 with L 15 at the P2 position, MDPTISSHD 9 TESTPL 15 N↓ETGHPNCTPILT, consistent with the site-directed mutagenesis approach above. Substituting arginine for leucine [13] completely eliminated the response to cat S ( Table 1 ; Fig. 5b ). Papain preferred L 15 at the P2 position and cleavage between N 16 and E 17 but no additional specificity was apparent, and cleavage otherwise occurred at multiple sites. 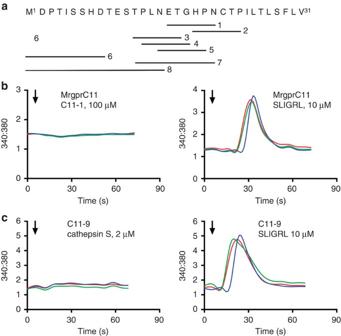Figure 5: N-terminal peptides do not activate MrgprC11 and cat S requires L15for activity. (a) A series of eight MrgprC11 N-terminal peptides was generated based on possible protease cleavage sites. (b) Calcium imaging of HeLa cells transfected with MrgprC11 following treatment with a representative MrgprC11 N-terminal peptide, C11-1 100 μM, the hexapeptide tethered ligand ETGHPN at the cat S cleavage site. (c) Cat S does not activate the MrgprC11 in which L15has been changed to R. Note that SLIGRL activates the native and mutant receptors. Arrows represent addition of test reagent. Figure 5: N-terminal peptides do not activate MrgprC11 and cat S requires L 15 for activity. ( a ) A series of eight MrgprC11 N-terminal peptides was generated based on possible protease cleavage sites. ( b ) Calcium imaging of HeLa cells transfected with MrgprC11 following treatment with a representative MrgprC11 N-terminal peptide, C11-1 100 μM, the hexapeptide tethered ligand ETGHPN at the cat S cleavage site. ( c ) Cat S does not activate the MrgprC11 in which L 15 has been changed to R. Note that SLIGRL activates the native and mutant receptors. Arrows represent addition of test reagent. Full size image MrgprC11 is not activated by tethered or diffusible ligands As conventional PARs are activated by tethered ligands generated following protease-mediated cleavage of their N-terminal domains, we sought to determine whether such peptides could activate MrgprC11. We generated a series of eight peptides ( Fig. 5a ; Supplementary Table 2 ) ranging from 6 to 15 amino acids based on predicted cleavage sites near the MrgprC11 N terminus. These included the tethered hexapeptide ETGHPN that begins at the cat S cleavage site, and the diffusible peptide MDPTISSHDTESTPLN that begins at the N terminus of MrgprC11 and ends at the cat S cleavage site. In contrast to PAR2 N-terminal peptides, synthetic MrgprC11 N-terminal peptides failed to elicit calcium responses in MrgprC11-expressing cells ( Fig. 5b ; Supplementary Fig. 2). These data reveal that in contrast to the activation of PARs, Mrgpr activation does not occur via generation of either a tethered or diffusible ligand. Proteases activate β2AR and MC1R–MrgprC11 hybrid receptors We have shown thus far that protease-mediated cleavage of MrgprC11 causes receptor activation without the formation of either a tethered or diffusible ligand. Another possible explanation of the ability of cysteine proteases to activate Mrgprs is that proteolysis of the extracellular domain results in a direct conformational change of the intracellular portion of the receptor that allows G-coupled signalling to occur. If this is the case, a mutant MrgprC11 in which the native N terminus has been substituted with the N terminus of an unrelated GPCR that can also be cleaved by cysteine proteases might be activated by proteolysis. To evaluate this possibility, we substituted the N terminus of MrgprC11 with either that of the β2-adrenergic receptor (β2AR) or the melanocortin-1 receptor (MC1R). These receptors are class A GPCRs, such as Mrgprs, but they couple primarily to Gs. We selected β2AR and MC1R because of the deep knowledge surrounding their structure and function. Each of these receptors contains residues that can be cleaved by cysteine proteases. However, biogenic amines and melanocortins, respectively, not proteases, are their conventional ligands. As predicted, both cat S and papain treatment of HeLa cells transfected with hybrid receptors β2AR–MrgprC11 or MC1R–MrgprC11 resulted in robust calcium signalling. As controls, protease treatment did not result in calcium mobilization in HeLa cells expressing native β2AR or MC1R ( Fig. 6 ). Taken together with the site-specific mutagenesis results, these findings argue that cat S- or papain-mediated cleavage of specific N-terminal residues directly triggers conformational changes in the transmembrane and/or intracellular domains of the MrgprC11 receptor that lead to downstream signalling. 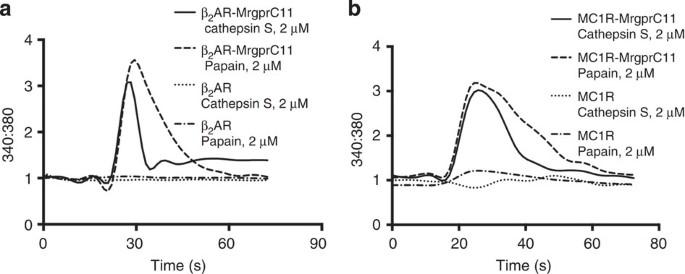Figure 6: Cathepsin S and papain activate MrgprC11 downstream signalling in N-terminal exchange receptors. (a) Cat S and papain activate β2AR–MrgprC11 but not the WT AR as determined by calcium imaging. (b) Cat S and papain activate MC1R–MrgprC11 but not WT MC1R as determined by calcium imaging. SeeSupplementary Fig. 4for additional details. Figure 6: Cathepsin S and papain activate MrgprC11 downstream signalling in N-terminal exchange receptors. ( a ) Cat S and papain activate β2AR–MrgprC11 but not the WT AR as determined by calcium imaging. ( b ) Cat S and papain activate MC1R–MrgprC11 but not WT MC1R as determined by calcium imaging. See Supplementary Fig. 4 for additional details. Full size image Effect of cysteine proteases on other Mrgprs To determine whether cysteine protease-mediated receptor activation was specific to MrgprC11, we examined whether cat S and papain were capable of triggering calcium mobilization in HeLa cells transfected with other members of the Mrgpr family, including human MRGPRX1–4 as well as mouse MrgprA3, which mediates chloroquine-induced itch. We found that in addition to activating human PAR2 and mouse MrgprC11, cat S activated human MRGPRX2 ( Table 2 ; Supplementary Fig. 5 ). Cat S failed to activate other human MRGPRs and mouse MrgprA3 ( Table 2 ). In contrast, papain activated human MRGPRX1, but had no effect on the other human MRGPRs ( Table 2 ; Supplementary Fig. 5 ). As expected, trypsin failed to activate these Mrgprs ( Fig. 2a ; Table 2 ). These results demonstrate that cysteine proteases activate only select Mrgprs, and that cat S, in particular, activates mouse and human Mrgprs that have been implicated in itch transmission. Table 2 Responses of PAR2 and Mrgprs following treatment with cat S, papain and trypsin as determined by calcium imaging. Full size table Endogenous and exogenous proteases have long been implicated in the pathogenesis of many inflammatory diseases, including skin diseases [9] , [10] , [18] , [19] .Our previous work showed that endogenous cat S and other proteases trigger histamine-independent itch [9] , [10] , [11] . Transgenic mice in which cat S is overexpressed spontaneously develop an intensely pruritic, eczematous disorder resembling atopic dermatitis [14] . In addition, cat S levels are selectively upregulated in psoriatic keratinocytes [19] , a condition also associated with considerable itch [20] , [21] , [22] . Intradermal injection of cat S elicits acute itch in human subjects as well as scratching in mice [11] , [14] . Until now, the exact mechanism by which cysteine proteases induce itch remained elusive and was presumed to require activation of the PAR2 receptor via generation of KVDGTS, a tethered ligand distinct from SLIGRL [17] . We demonstrate for the first time that the cysteine proteases cat S and papain directly activate MrgprC11 to evoke histamine-independent scratching behaviour. The activation kinetics of MrgprC11 by papain were prolonged relative to that of cat S. The mechanism for this prolonged activation is not clear but may result from a balance of receptor activation/inactivation, calcium-induced release from intracellular stores or perhaps endosomal receptor signalling associated with papain [23] , [24] . Consistent with protease activation of MrgprC11, scratching responses elicited by the intradermal injection of cat S were significantly reduced in Mrgpr cluster Δ −/− mice, but remained intact in PAR2 −/− mice. In vitro correlates of these in vivo observations were demonstrated as the capacity of cat S to activate DRG neurons from Mrgpr cluster Δ −/− mice was markedly diminished while not significantly diminished in PAR2 −/− DRG neurons. RNAi knockdown of MrgprC11 specifically abolished the response of DRG neurons to cat S. In contrast, knockdown of MrgprA3 did not diminish the response of DRG neurons to cat S. It is not clear why the decrease in scratching responses in Mrgpr cluster Δ −/− mice, while significant, was not as substantial as the decrease in Ca ++ signals in DRG neurons from these mice. An explanation is that cat S activates PAR2 on keratinocytes, resulting in the release of thymic stromal lymphopoietin, a skin-derived cytokine that has been shown to induce itch via neuronal receptors for this molecule [25] . In addition, while PAR2 does not appear to have a direct role in cat S-evoked itch in WT mice, a non-native role may be unmasked in the absence of MrgprC11. Our data also identify the cysteine protease cat S as a functional endogenous ligand for Mrgprs, currently considered as orphan receptors. Whether other endogenous cysteine proteases activate Mrgprs awaits future investigations. Conventional PARs are GPCRs that are uniquely activated by proteolysis. In this scenario, proteases bind and specifically cleave residues in the N-terminal domain of the receptor to unmask a ‘tethered’ ligand that subsequently interacts with another portion of the receptor to trigger intracellular signalling. Similarly, PARs can be activated by synthetic hexapeptides that mimic the first six amino acids of the unmasked N terminus. The data presented here are the first to demonstrate that GPCRs other than PARs can be activated by proteolysis, as cysteine proteases activate MrgprC11. Site-specific mutagenesis revealed that cat S requires L 15 and papain requires D 9 and L 15 for cleavage, while data from MS/MS demonstrated that cleavage occurs between residues N 16 and E 17 . In contrast to PARs, tethered ligands do not appear to play a role in Mrgpr activation, and synthetic Mrgpr N-terminal peptides have no apparent functional activity. These data highlight the possibility that cysteine proteases may exert effects on other ‘non-PAR’ GPCRs and further suggest that proteases are capable of modulating GPCRs by multiple mechanisms. Classically, GPCRs are thought to become activated when ligands bind in a pocket formed by the transmembrane helices thereby triggering exposure of cytoplasmic domains required for coupling to heterotrimeric G-protein subunits [26] . PARs, on the other hand, become activated when proteolysis allows for tethered ligands to interact with residues in the second extracellular wloop, subsequently resulting in conformational changes in the transmembrane helices [16] , [17] . While the exact mechanism by which proteolysis triggers activation of MrgprC11 remains unknown, we suggest that the N-terminal domain interacts with the extracellular loops of the receptor to lock it in an inactive state. Cleavage of the N terminus by cysteine proteases may release this lock, shifting transmembrane and cytoplasmic domains as suggested with traditional PARs. Our observations that calcium signalling was evoked by cathepsin-induced proteolysis of the β2AR and MC1R N-terminal exchange mutants are consistent with this hypothesis. The mechanism underlying this observation deserves further study. It is interesting that although N-terminal MrgprC11 peptides did not activate Mrgpr signalling, SLIGRL, a PAR2 N-terminal peptide, is capable of inducing itch via activation of MrgprC11 (ref. 3 ), at least at micromolar concentrations. Whether this effect occurs naturally is not clear. The concept that N-terminal peptides released into the extracellular milieu following PAR cleavage may exert a biologic effect independent of PARs has been reported. PAR1 cleavage by thrombin generates an N-terminal peptide known as parstatin, which is capable of inhibiting vascular endothelial cell growth factor- and fibroblast growth factor-induced angiogenesis in vitro and in vivo . It also plays a role in modulating platelet function [27] , [28] . Whether protease-mediated cross-signalling between PAR2 and MrgprC11 serves a relevant role in coupling itch and inflammation in vivo is not known. Cysteine proteases, in particular cysteine cathepsins, are widely expressed in mammalian tissues and have been implicated in the pathophysiology of a diverse array of inflammatory, autoimmune and allergic diseases, as well as in neuropathic pain [15] , [29] , [30] , [31] , [32] . Recent work in murine colitis models demonstrates that macrophage- and microglial cell-derived cat S induces colonic inflammation and pain by activating PAR2 on different cell types, linking increased paracellular permeability in colonocytes with nociceptive hyper-excitability and neurogenic inflammation in primary spinal afferent neurons [15] , [33] , [34] , [35] . We suggest that cat S may similarly act as a key regulator linking itch and inflammation in the skin. Our work reveals a novel mechanism by which cat S accomplishes its diverse effects: activation of MrgprC11. Increased cat S expression has been reported in several common inflammatory skin conditions, including atopic dermatitis, psoriasis and seborrhoeic dermatitis [14] , [19] , [36] . Under these conditions, cat S may simultaneously contribute to itch and propagate inflammation via different but related mechanisms. First, as we demonstrated here, cat S induces itch directly by activating MrgprC11. Second, cat S-mediated activation of PAR2 may induce itch if PAR2 N-terminal peptides bind to MrgprC11 on primary sensory nerves. In addition, PAR2 activation in keratinocytes may trigger the release of thymic stromal lymphopoietin, which in turn activates cutaneous sensory neurons that express transient receptor potential ankyrin channel A1 (TRPA1), leading to itch stimulation and neurogenic inflammation [25] . Recognizing that proteases can recruit multiple distinct pathways to induce itch and inflammation may help drive the development of more effective therapeutic strategies to treat inflammatory diseases, shifting the focus from blocking individual downstream receptors to inhibiting protease–receptor complexes. Reagents, peptides and antibodies Recombinant cat S was generated as previously described [11] , [17] and diluted in 1 × PBS, pH 7.4, 5 mM EDTA, 5 mM dithiothreitol and 5 mM cysteine chloride. Papain (Sigma-Aldrich) was diluted in 0.1 × PBS, 50 mM sodium acetate, pH 6.5, 5 mM EDTA, 5 mM dithiothreitol and 5 mM cysteine chloride. Crystalline papain is more active and has a broader cleavage range than recombinant cat S. Different incubation times or concentrations were thus used as indicated. N-terminal peptides derived from the sequence of MrgprC11 were obtained from GenScript and diluted in PBS. The 28 amino-acid N-terminal peptide MDPTISSHDTESTPLNETGHPNCTPILT was made by Peptide 2.0 (Chantilly, VA). The cysteine protease inhibitor E-64 was obtained from Sigma-Aldrich. Similar results were obtained at either 5 or 10 μM of this compound. Anti-Gaussia luciferase, catalogue # E8023S from New England Biolabs was used at a dilution of 1:1,500. Anti-phospho-PKC (pan) (βII Ser660) catalogue #9371 from Cell Signaling Technology was used at a dilution of 1:1,000. Horseradish peroxidase (HRP)-labelled donkey anti-rabbit, catalogue # NB660–894, and anti-mouse antibodies, catalogue # NB7544, were from Thermo Fisher and used at 1:2,000 and 1:5,000, respectively. Molecular weight markers were Bioreagents EZ-run prestained rec protein ladder, cat # 3603500 from Thermo Fisher. All other reagents were purchased from Invitrogen, unless otherwise noted. Mice WT and PAR2 KO mice were obtained from Jackson Laboratories. Mrgpr cluster Δ −/− mice were generated by X.D. as previously described [2] . The mouse studies were performed at Johns Hopkins and approved by the IACUC at that institution. Cell culture HeLa cells were obtained from the ATCC and maintained in DMEM supplemented with fetal bovine serum, L -glutamine, penicillin and streptomycin (Fisher Biochemicals). Dissociated DRG neurons were prepared from WT, Mrgpr cluster Δ −/− , PAR2 −/− and Pirt-GCaMP3 mice as reported previously [2] . DRGs were collected from all spinal levels of 4-week-old mice, placed in cold medium and treated with enzyme solution at 37 °C. Following titration and centrifugation, cells were suspended, plated on glass coverslips coated with poly- D -lysine and laminin, incubated at 37 °C and used within 48 h. Cloning of WT MrgprC11 and generation of mutants The coding region of MrgprC11 was cloned by PCR from mouse genomic DNA using the forward and reverse primers: 5′-GCGCTCGAGAGCATGGATCCAACCATCTCATC-3′ and 5′-GCGAAGCTTTCAATATCTGCTTTCTGAAATCTC-3′. C11 N-terminal mutants were made by site-specific mutagenesis procedures using the primer pairs listed in Supplementary Table 3 to change the listed residues to isoleucine or arginine at the P2 site. Leucine at P2 is the preferred site for cleaved by cathepsin S as in native MrgprC11, with isoleucine less so and arginine not at all. Preparation of G. luciferase –MrgprC11 fusion cDNAs G. luciferase complementary DNA (cDNA) was cloned, without its termination codon, into pcDNA3.1(−) as an XbaI–XhoI fragment. MrgprC11 cDNA was fused as an XhoI–HindIII unit at the 3′ terminus of the luciferase cDNA to obtain LucMrgprC11. Preparation of MrgprC11 with β2AR and MC1R amino termini The MrgprC11-coding region without its N terminus from amino-acid 34 to its C terminus was cloned as an EcoRI–HindIII cDNA into pcDNA3.1(−) to obtain the vector pMrgprC11NR. The N termini of β2AR and MC1R from amino acids 1–34 and 1–37, respectively, were isolated as XhoI–EcoRI fragments by PCR, and cloned into pMrgprC11NR to generate the vectors pARC11 and pMC1RC11 for expression of the chimeric receptors β2AR–MrgprC11 and MC1R–MrgprC11. Calcium imaging HeLa cells were grown to confluence, trypsinized and then transfected with the pcDNA vector carrying the G. luciferase– MrgprC11 fusion construct, MrgprC11 cDNA or salmon sperm DNA as a control using Lipofectamine 2000. Transfected cells were plated into 96-well glass-bottom plates at 50,000 cells per well and maintained at 37 °C in 5% humidified CO 2 for 3 h after which time the medium was replaced. Twenty-four to 48 h after transfection, cells were incubated for 60 min at room temperature with 2 μM of Fura-2-acetoxymethyl ester (Fura-2) diluted in complete DMEM. Following Fura-2 loading, the medium was replaced with 90 μl of HEPES-buffered saline (20 mM HEPES, 115 mM NaCl, 5.4 mM KCl, 2 mM CaCl 2 , 0.8 mM MgCl 2 and 13.8 mM glucose, pH 7.4) and cells were used immediately for calcium imaging. A luciferase–receptor construct was used in all tranfections to establish consistency of transfection efficiency. Ratiometric calcium imaging was performed using a Zeiss Axiovert 200 M microscope equipped with a flipping filter wheel and Axiovision software (version 4.6). Peptide and protease agonists, cat S or papain (10 μl) were added 15 s after initiating image acquisition and typically represented by down arrows in the figures. Images were acquired at time 0 and every 5 s thereafter for at least 90 s. All images obtained during each acquisition period were analysed. Each experiment was performed at least three times, and ratiometric changes were measured in at least 20 cells per acquisition with responses of three representative cells depicted in the figures in the Results or Supplementary Information . Primary DRGs cultured from WT, Mrgpr cluster Δ −/− and PAR2 −/− mice were loaded with Fura-2 for 30 min at 37 °C for ratiometric calcium imaging as described above following application of cat S and papain (5 and 20 μM, respectively). For experiments incorporating RNA interference, MrgprA3 and MrgprC11 on-target short interfering RNAs (siRNAs) were purchased from Thermo Scientific. MrgprA3 or MrgprC11 siRNA (0.175 nmol) were electroporated, respectively, into DRG neurons from Pirt-GCaMP3 mice that had been generated previously [2] , [37] . Electroporation of dissociated DRG neurons with Mrgpr-expression constructs was carried out using Mouse Neuron Nucleofector Kit (Amaxa Biosystems) following the manufacturer’s instructions. Electroporated neurons were plated and cultured as described above and used within 72 h. Green fluorescence from genetically encoded calcium GCaMP3 was detected via single-photon Ca2+ imaging with a 700 Zeiss confocal microscope, using the 488-nm line of a solid-state laser for excitation of Pirt-GCaMP3 and a 488-nm laser main dichroic beam splitter and a 505–555-nm variable secondary dichroic mirror to detect the emission of green fluorescence. Real-time quantitative PCR Total RNA was extracted from cultured DRGs 3 days after siRNA electroporation using an Rneasy micro kit (Qiagen). Purified RNA was quantified on a Nanodrop 2000 UV spectrophotometer (Thermal Scientific) at 260 nm and assessed for purity using the 260/280-nm ratio. DNA was reverse transcribed with the Superscript First Strand Synthesis System (Invitrogen). PCR amplifications were carried out with a Step One Plus real time PCR system (Applied Biophysics). PCR conditions were 95 °C for 3 min and 50 cycles of 95 °C for 30 s and 60 °C for 60 s. Primers as listed below: MrgprC11-F 5′-AGCATCCACAACCCCAGAAG-3′; MrgprC11-R 5′-TGGAGTGCAGTTGGGATGAC-3′; MrgprA3-F 5′-ACACAAGCCAGCAAGCTACA-3′; MrgprA3-R 5′-ACTTCCAGGGATGGTTTCGT-3′; Actin-F 5′-CGTCGACAACGGCTCCGGCATG-3′; Actin-R 5′-CCACCATCACACCCTGGTGCCTAGG-3′ All primers were intron spanning to avoid genomic DNA contamination. Melting curve analysis was applied to all final PCR products after the cycling protocol. Samples were run in triplicate, and threshold cycle (Ct) values from each reaction were averaged. Relative messenger RNA levels of MrgprA3 and MrgprC11 were calculated from threshold cycles and normalized to the actin level. Experiments were carried out three times with samples from different animals, and the Student’s t -test was used to determine significance. Concentration-effect measurements for cat S and papain HeLa cells transfected with MrgprC11 cDNA were analysed using ratiometric imaging as described above with cat S and papain at concentrations from 1 nM to 10 μM. Each of the concentration-dependent readings was performed in triplicate. Maximum intensities at each of the dilutions were calculated and plotted against concentration using GraphPad Prism software. Error bars represent s.e.m. within an experiment, although these experiments were performed multiple times with similar results. Luciferase assay MrgprC11 plasmid DNA (10 μg) or salmon sperm as control was transfected into 2 × 10 6 HeLa cells as described above and plated into 10-cm dishes. Forty-eight hours after transfection, the cells were washed with PBS, scraped and pelleted. Cells were suspended in a volume of 200 μl PBS and 100 μl were incubated with cat S (2 μM) or papain (0.02 μM) in the presence or absence of the irreversible cysteine protease inhibitor E-64 for 10 min at room temperature. Control cells were not treated with protease. Protease activity was quenched by adding 300 μl of complete DMEM, after which the cells were centrifuged and supernatants (50 μl) were assayed in triplicate for luminescence according to the instructions of the manufacturer (New England Biolabs). These experiments were performed multiple times with protease activity being quenched at many different time points so as to catch luminescence associated with papain, as this protease has the capacity to digest luciferase. Western blot analysis for luciferase HeLa cells transfected with the G. luciferase– MrgprC11 fusion construct were treated with cat S (2 μM) or papain (0.02 μM) for 10 min. Cells were pelleted and the supernatant was added directly to loading buffer to quench enzymatic activity, run on NuPAGE Novex Bis-Tris mini gels and transferred to nitrocellulose membranes. Membranes were probed with a primary rabbit anti- G. luciferase antibody followed by HRP-labelled donkey anti-rabbit antibody for reaction with the ECL substrate to identify protein bands. The results presented are representative of one of four experiments. Western blot analysis for p-PKC (Ser660) HeLa cells were transfected with MrgprC11 plasmid DNA as described above and plated onto three 10-cm dishes. Non-transfected HeLa cells were also plated into three other 10-cm dishes. Forty-eight hours after transfection, cells were washed with PBS and then treated with papain or cat S at 0.02 and 2 μM, respectively, for 10 min. A subset of HeLa cells that were not transfected was treated with papain, cat S or PBS alone as controls. Cells were harvested by scraping, pelleted and lysed by repetitive freeze–thaw cycles. Cell lysates were centrifuged at 4 °C for 15 min. Supernatants were collected and protein concentrations were determined by the Bradford assay. Equal amounts of cell lysates were loaded onto NuPAGE Novex Bis-Tris mini gels, electrophoresed and transferred to nitrocellulose membranes. Membranes were probed with rabbit anti-phospho-PKC (βII Ser660) followed by incubation with HRP-labelled donkey anti-rabbit antibody for reaction with the ECL substrate to identify protein bands on the membrane. The blot was re-probed with mouse anti-actin antibody to identify the control actin band (42 kDa). HRP-labelled anti-mouse antibody was used as a secondary antibody for the ECL substrate. This experiment was repeated three times and error bars represent ±s.e.m. between the individual bands between three separate experiments, with relative intensities quantified using ImageJ. Behavioural studies All mice used for behavioural studies were 2- to 3-month-old males (20–30 g) and were backcrossed to C57BL/6 mice for at least 10 generations. Mice were habituated for 30 min per day for 3 days prior and then at least 15 min on the day of the study. Intradermal injections of 10 μl cat S 80 μM were delivered to the cheek [13] . Scratching behaviour was observed for 30 min. A scratching bout was defined as continuous scratching movements with hind paws directed at the site of injection. Scratching behaviour was quantified by recording the number of scratching bouts at 5-min intervals over a 30-min observation period. Experimenters were blind to genotype. Data are presented as mean±s.e.m. n represents the number of mice analysed or times the experiments were performed. The distribution of the variables in each experimental group was approximately normal. Statistical comparisons were conducted by two-tailed, unpaired Student’s t -test. Differences were considered to be statistically significant for P <0.05. Representative data are from experiments that were replicated biologically at least three times with similar results. How to cite this article: Reddy, V. B. et al. Redefining the concept of protease-activated receptors: cathepsin S evokes itch via activation of Mrgprs. Nat. Commun. 6:7864 doi: 10.1038/ncomms8864 (2015).